The TORC1 effector kinase Npr1 fine tunes the inherent activity of the Mep2 ammonium transport protein The TORC1 complex controls cell growth upon integrating nutritional signals including amino-acid availability. TORC1 notably adapts the plasma membrane protein content by regulating arrestin-mediated endocytosis of amino-acid transporters. Here we demonstrate that TORC1 further fine tunes the inherent activity of the ammonium transport protein, Mep2, a yeast homologue of mammalian Rhesus factors, independently of arrestin-mediated endocytosis. The TORC1 effector kinase Npr1 and the upstream TORC1 regulator Npr2 control Mep2 transport activity by phospho-silencing a carboxy-terminal autoinhibitory domain. Under poor nitrogen supply, Npr1 enables Mep2 S457 phosphorylation and thus ammonium transport activity. Supplementation of the preferred nitrogen source glutamine leads to Mep2 inactivation and instant S457 dephosphorylation via plasma membrane Psr1 and Psr2 redundant phosphatases. This study underscores that TORC1 also adjusts nutrient permeability to regulate cell growth in a fast and flexible response to environmental perturbation, establishing a hierarchy in the transporters to be degraded, inactivated or maintained active at the plasma membrane. TOR (target of rapamycin) is a conserved serine/threonine kinase forming two functionally distinct complexes (TORC1 and TORC2) and controlling cell growth upon integration of environmental cues such as nutritional availability and energy status inputs. In mammalian cells, mTORC signalling regulates key processes such as protein synthesis and autophagy and is involved in an increasing number of pathological outcomes including cancer, type-2 diabetes and neurodegeneration [1] . Emerging concepts link yeast TORC1 and arrestin-like adaptors in the modulation of the composition of plasma-membrane proteins via ubiquitin-mediated endocytosis of transporters in response to nutrient availability [2] , [3] . The Npr1 (nitrogen permease reactivator 1) kinase is a TORC1 effector responding to the quality of the nitrogen supply and controlling the stability of nitrogen source transporters [4] , [5] . During poor nitrogen supply or rapamycin treatment, namely under conditions that downregulate TORC1, Npr1 is weakly phosphorylated and assumed to be active, while the presence of a preferred nitrogen source leads to increased phosphorylation of Npr1 and to theoretical inactivation of the kinase [4] , [6] , [7] . Npr1-dependent phosphorylation of arrestin-like proteins prevents recruitment of the Rsp5 ubiquitin-ligase to its plasma-membrane targets, thus protecting them from ubiquitylation, endocytosis and lysosomal degradation [2] , [3] . With glutamine and asparagine, ammonium is a preferred nitrogen source for yeast cells. Ammonium also serves as principal nitrogen source for numerous microorganisms and plants, whereas it is mainly regarded as a blood pH regulator and a cytotoxic compound in mammals [8] , [9] , [10] . Three Mep-Amt proteins enable ammonium transport in Saccharomyces cerevisiae [11] . These belong to the Mep-Amt-Rh protein superfamily, including the human Rhesus (Rh) blood group antigens and mediating ammonium transport in organisms as distant as bacteria and mammals [12] , [13] , [14] . Available x-ray structures of Mep-Amt-Rh proteins reveal a similar trimeric fold, with a conducting pore crossing each of the three monomers [15] , [16] , [17] , [18] , [19] , [20] . One monomer comprises 11 or 12 helices and is prolonged by a cytosolic C-terminal extension of variable length. Among yeast Mep-Amt proteins, Mep2 has a proposed additional signalling role in the induction of filamentation during ammonium deprivation and in the nutrient-responding PKA pathway [21] , [22] . While studying how proteins transporting favoured nitrogen sources are regulated, we found that Npr1 is required for the activity of all three Mep-Amt proteins but the underlying mechanism remained unsolved [23] , [24] . Focusing on Mep2, this study reveals that the TORC1 effector Npr1 does not control arrestin-mediated endocytosis of the transport protein. Instead, the kinase fine tunes the Mep2 activity by controlling the phosphorylation of an autoinhibitory domain in the cytosolic C-terminal extension. We identify two plasma membrane phosphatases involved in Mep2 activity tuning, as well as an upstream regulator of the TORC1 signal to Mep2. Thus, TORC1 not only triggers endocytosis of nutrient transporters but also tunes the inherent activity of plasma-membrane targets to control cell growth. Mep2 is phosphorylated in an Npr1-dependent manner During growth in the presence of a nonpreferred nitrogen source, Mep2 is highly produced and active in wild-type cells whereas the Mep2 transport activity is completely lost in cells lacking the Npr1 kinase [24] . We first checked the influence of Npr1 on the stability of Mep2 in this growth condition and unexpectedly found that Mep2 is not destabilized in Npr1-lacking cells ( Fig. 1a ). Yet, in wild-type cells, the Mep2 monomer is detected as a doublet of two major bands separated by a ~6–8 kDa shift, whereas it appears as one major intense and low-molecular-weight form in Npr1-lacking cells. As native Mep2 is heavily glycosylated, the membrane protein extracts for this experiment were treated with N -glycosidase before SDS–PAGE. Similar results were obtained upon immunodetection of the non-glycosylable version Mep2 N4Q expressed in triple- mepΔ cells lacking the three endogenous MEP genes ( Fig. 1b ). This Mep2 version will be used in following experiments, as it has the advantage of migrating as discrete bands on a gel while retaining the major properties of native Mep2 (ref. 25) [25] . Expression of a plasmidic MEP2 version in the triple- mepΔ background context will further enable to specifically assess the Mep2 functionality. 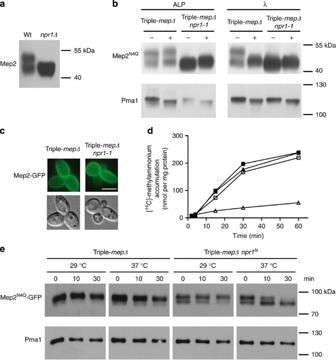Figure 1: Npr1-dependent phosphorylation of Mep2 correlates with transport activity. (a) Immunodetection of Mep2 from membrane-enriched cell extracts treated withN-glycosidase F. Wild-type (23344c) andnpr1Δ(30788a) cells were grown with proline (0.1%) as sole nitrogen source. (b) Immunodetection of Mep2N4Qfrom membrane-enriched extracts treated (+) or not (−) with alkaline (ALP) orλphosphatase. Triple-mepΔ(31019b) and triple-mepΔ npr1-1(31052c) cells transformed with YCpMep2N4Qwere grown with proline (0.1%). The plasma membrane proton ATPase Pma1 was detected as loading and phosphatase treatment controls. (c) Mep2-GFP localization was observed by fluorescence microscopy in triple-mepΔ(31019b) and triple-mepΔ npr1-1(31052c) cells transformed with pGAL1Mep2-GFP and grown with proline (0.1%) and galactose (3%) plus glucose (0.3%). Scale bar, 5 μm. (d) [14C]-methylammonium (0.5 mM) accumulation by Mep2N4Q-GFP expressed from triple-mepΔ(31019b, squares) and triple-mepΔ npr1ts(MB063, triangles) cells after transfer at 29 °C (black symbols) or 37 °C (white symbols). Cells were transformed with pGAL1Mep2N4Q-GFP and grown with proline (0.1%). (e) Immunodetection of Mep2N4Q-GFP from total extracts of cells collected after the temperature shift described inFig. 1d. Pma1 was detected as a loading control. Figure 1: Npr1-dependent phosphorylation of Mep2 correlates with transport activity. ( a ) Immunodetection of Mep2 from membrane-enriched cell extracts treated with N -glycosidase F. Wild-type (23344c) and npr1Δ (30788a) cells were grown with proline (0.1%) as sole nitrogen source. ( b ) Immunodetection of Mep2 N4Q from membrane-enriched extracts treated (+) or not (−) with alkaline (ALP) or λ phosphatase. Triple- mepΔ (31019b) and triple- mepΔ npr1-1 (31052c) cells transformed with YCpMep2 N4Q were grown with proline (0.1%). The plasma membrane proton ATPase Pma1 was detected as loading and phosphatase treatment controls. ( c ) Mep2-GFP localization was observed by fluorescence microscopy in triple- mepΔ (31019b) and triple- mepΔ npr1-1 (31052c) cells transformed with pGAL1Mep2-GFP and grown with proline (0.1%) and galactose (3%) plus glucose (0.3%). Scale bar, 5 μm. ( d ) [ 14 C]-methylammonium (0.5 mM) accumulation by Mep2 N4Q -GFP expressed from triple- mepΔ (31019b, squares) and triple- mepΔ npr1 ts (MB063, triangles) cells after transfer at 29 °C (black symbols) or 37 °C (white symbols). Cells were transformed with pGAL1Mep2 N4Q -GFP and grown with proline (0.1%). ( e ) Immunodetection of Mep2 N4Q -GFP from total extracts of cells collected after the temperature shift described in Fig. 1d . Pma1 was detected as a loading control. Full size image We next tested whether the two Mep2 forms detected in wild-type cells correspond to differentially phosphorylated states of the protein. Phosphorylation can alter the migration profile of a protein during SDS–PAGE in different ways according to the effect of phosphate on the local charge and on SDS coating [26] . Treating protein extracts with alkaline phosphatase (ALP) did not lead to a removal of the Mep2 N4Q slower-running form ( Fig. 1b ). ALP treatment did, however, cause a slight upshift (~1–2 kDa) of both Mep2 N4Q bands. A similar upshift was also detected on the major Mep2 N4Q form in Npr1-lacking cells. These data indicate that both Mep2 forms are phosphorylated in wild-type cells. This is also the case of the unique form detected in the npr1 mutant, suggesting that this phosphorylation event is Npr1 independent. Nevertheless, treatment with the lambda ( λ ) phosphatase caused a complete conversion of the slower-running Mep2 N4Q form into a faster-running one ( Fig. 1b ). In Npr1-lacking cells, the λ phosphatase treatment led to an upshift of the major Mep2 N4Q form, as observed with ALP treatment. The slower-running form of Mep2 in wild-type cells results from a major phosphorylation event, Npr1 dependent, whereas both fast and slow-running Mep2 forms are targeted by another phosphorylation event, a minor phosphorylation, Npr1 independent. The Npr1-dependent phosphorylated site(s) of Mep2 appear(s) highly resistant to dephosphorylation by ALP while sensitive to λ phosphatase treatment. For simplification, the Npr1-dependent and slower-running form of Mep2 will be called the phosphorylated form of the protein. Fluorescence microscopy revealed that Npr1 is dispensable for proper cell surface localization of Mep2-GFP ( Fig.1c ). Further supporting a plasma membrane insertion of Mep2 in the absence of a functional Npr1 kinase, proteolytic shaving of Npr1-lacking protoplasts showed accessibility of the periplasmic N -glycosylated amino terminus of Mep2 to enzymatic digestion ( Supplementary Fig. 1 ). Hence, Npr1 is required for Mep2 inherent transport activity and is associated with the immunodetection of a phosphorylated form, possibly representing an active state of the transport protein. Npr1 inactivation correlates with Mep2 inactivation We next used cells expressing a thermosensitive Npr1 variant [27] to test the consequence of immediate Npr1 inactivation on the transport activity and the migration profile of plasma membrane Mep2 ( Fig. 1d,e ). A MEP2 gene controlled by the galactose-inducible GAL1 promoter was used to produce Mep2 in galactose-growing cells. Glucose was then added for 90 min to stop MEP2 transcription and allow accumulation of Mep2 at the plasma membrane. At this stage, inactivation of the Npr1 kinase by shifting npr1 ts cells at 37 °C strongly reduced the Mep2-dependent accumulation of [ 14 C]-methylammonium (mea), a convenient tracer analogue of ammonium ( Fig. 1d ). This is consistent with Mep2 inherent activity largely relying on the maintenance of the kinase integrity. Inactivation of Npr1 was also accompanied by a rapid fading of the Mep2 phosphorylated form with a concomitant intensification of the faster-running one ( Fig. 1e ), revealing a rapid Mep2 dephosphorylation linked to Npr1 inactivation. A similar behaviour of Mep2 was observed when the experiment was performed with end3 npr1 ts cells, further altered in endocytosis ( Supplementary Fig. 2 ). These data indicate that plasma membrane Mep2 is sensitive to a phosphatase activity likely involved in its inactivation. The Npr1 integrity appears necessary at the plasma membrane to maintain the phosphorylated Mep2 form and keep Mep2 active. Npr1 controls Mep2 activity via S457 phosphorylation We used the NetPhosYeast 1.0 server ( http://www.cbs.dtu.dk/services/NetPhosYeast/ ) to predict putative phosphorylation sites in Mep2. Among the cytosolic candidates, S227 lies at the limit of intracellular loop (IL) 3 and transmembrane helix (TM) 6, whereas all other are in the C-terminal tail (S426, S457, T459, S460, S484, T485, S487, S490, S491, T495). Two large-scale mass spectrometry analyses revealed at least four phosphorylated sites (S484, S487, S490, S491) in the Mep2 C terminus, all of them responding to the addition of rapamycin [28] , [29] . We thus focused on the Mep2 C-terminal sites to unravel potential targets of the Npr1 regulation and first used site-directed mutagenesis to replace all seven last serines and threonines (S484, T485, S487, S490, S491, T492, T495) by alanines. However, the resulting Mep2 N4Q,7ST/A variant was still detected as a doublet band ( Supplementary Fig. 3a ). This was also the case for the S426A Mep2 variant (Mep2 N4Q,S426A ) ( Supplementary Fig. 3b ). Finally, we constructed a Mep2 variant bearing replacement into alanines of the three remaining candidate residues (Mep2 N4Q,S457A,T459A,S460A ). While Mep2 N4Q was detected as two forms, Mep2 N4Q,S457A, T459A,S460A was detected as one major form, likely lacking the Npr1-dependent phosphorylation ( Fig. 2a ). To precisely define the phosphorylated amino-acid target(s), double and single S/T-to-A Mep2 variants were constructed. Only the Mep2 N4Q,S457A,S460A variant was detected as one major form, indicating S457 and S460 as phosphorylated sites. λ phosphatase treatment revealed that the modification of Mep2 N4Q,S457A and Mep2 N4Q,S460A corresponds to a phosphorylation ( Supplementary Fig. 4 ). Each of the S457 and S460 residues was also replaced by the phosphomimetic aspartate residue. The resulting Mep2 N4Q,S457D and Mep2 N4Q,S460D variants migrated slower than Mep2 N4Q when considering extracts from cells containing Npr1 but also from Npr1-lacking cells ( Fig. 2a ), indicating that the presence of a negatively charged residue at these positions is sufficient to alter the migration behaviour of Mep2. 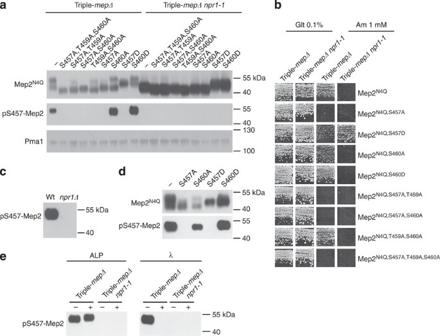Figure 2: Npr1 controls Mep2 activityviaS457 phosphorylation. (a,b) Triple-mepΔ(31019b) and triple-mepΔ npr1-1(31052c) cells were transformed with YCpMep2N4Q, YCpMep2N4Q,S457A,T459A,S460A, YCpMep2N4Q,S457A,T459A, YCpMep2N4Q,S457A,S460A, YCpMep2N4Q,T459A,S460A, YCpMep2N4Q,S457A, YCpMep2N4Q,S460A, YCpMep2N4Q,S457D, or with YCpMep2N4Q,S460D. (a) Immunodetection of total Mep2N4Qand S457-phosphorylated Mep2N4Q(pS457-Mep2) from membrane-enriched extracts of proline-grown cells. Pma1 was detected as a loading control. (b) Growth tests on solid medium containing, as the sole nitrogen source, 1 mM ammonium (Am) or 0.1% glutamate (Glt, positive growth control). Cells were incubated at 29 °C for 4 days. (c) Immunodetection of pS457-Mep2 using the same membrane as inFig. 1a. (d) Immunodetection of Mep2N4Qand pS457-Mep2 from membrane-enriched extracts of proline-grown triple-mepΔ(31019b) cells transformed with YCpMep2N4Q, YCpMep2N4Q,S457A, YCpMep2N4Q,S460A, YCpMep2N4Q,S457D, or with YCpMep2N4Q,S460D. (e) Immunodetection of pS457-Mep2 using the same membrane as inFig. 1b. Figure 2: Npr1 controls Mep2 activity via S457 phosphorylation. ( a , b ) Triple- mepΔ (31019b) and triple- mepΔ npr1-1 (31052c) cells were transformed with YCpMep2 N4Q , YCpMep2 N4Q,S457A,T459A,S460A , YCpMep2 N4Q,S457A,T459A , YCpMep2 N4Q,S457A,S460A , YCpMep2 N4Q,T459A,S460A , YCpMep2 N4Q,S457A , YCpMep2 N4Q,S460A , YCpMep2 N4Q,S457D , or with YCpMep2 N4Q,S460D . ( a ) Immunodetection of total Mep2 N4Q and S457-phosphorylated Mep2 N4Q (pS457-Mep2) from membrane-enriched extracts of proline-grown cells. Pma1 was detected as a loading control. ( b ) Growth tests on solid medium containing, as the sole nitrogen source, 1 mM ammonium (Am) or 0.1% glutamate (Glt, positive growth control). Cells were incubated at 29 °C for 4 days. ( c ) Immunodetection of pS457-Mep2 using the same membrane as in Fig. 1a . ( d ) Immunodetection of Mep2 N4Q and pS457-Mep2 from membrane-enriched extracts of proline-grown triple- mepΔ (31019b) cells transformed with YCpMep2 N4Q , YCpMep2 N4Q,S457A , YCpMep2 N4Q,S460A , YCpMep2 N4Q,S457D , or with YCpMep2 N4Q,S460D . ( e ) Immunodetection of pS457-Mep2 using the same membrane as in Fig. 1b . Full size image To test whether phosphorylation at S457 and/or S460 is required for the Mep2 function, growth tests were performed on a minimal solid medium containing a low ammonium concentration as sole nitrogen source ( Fig. 2b ). Triple- mepΔ cells, lacking or not a functional Npr1, and expressing Mep2 variants with all the combinations of the S457A, T459A and S460A mutations were assayed. In the presence of Npr1, only cells expressing Mep2 variants bearing at least the S457A substitution were unable to grow, suggesting that S457 phosphorylation is required for Mep2 function. Furthermore, cells expressing Mep2 N4Q,S457D were able to grow on low ammonium and this was true in the presence and absence of Npr1, indicating that the latter Mep2 variant shows a constitutive activity, independent of the kinase integrity. Growth tests conclusions were corroborated by measurements of initial uptake rates of [ 14 C]-methylammonium ( Table 1 ). Table 1 Methylammonium uptake activity of Mep2 variants. Full size table To ascertain that S457 is a direct target of phosphorylation and develop a tool to further study the regulatory events controlling Mep2 activity, a phospho-specific antiserum (pS457) was raised against a peptide centred on phosphorylated S457. In the presence of Npr1, the purified pS457 antibodies specifically recognized a Mep2 form with the same running rate as the phosphorylated slow-running Mep2 form ( Fig. 2a,c,d ). As expected, the S457-phosphorylated Mep2 form was not detected in Npr1-lacking cells or when using the Mep2 N4Q,S457A variant ( Fig. 2a,c,d ). It is to note that the Mep2 N4Q,T459A,S460A did not cross-react with pS457 antibodies, most probably due to alteration of the short antigenic recognition site by two simultaneous mutations ( Fig. 2a ). The phosphorylation at S457 was completely insensitive to ALP treatment whereas it was totally absent after λ phosphatase treatment ( Fig. 2e ). Hence, the S457 phosphorylation corresponds to the above-described Mep2 major phosphorylation, Npr1 dependent and ALP resistant. Npr1-dependent phosphorylation at S457 is thus required for Mep2 activity. Npr1 controls Mep2 conformation To get into the molecular mechanism of Npr1 control of Mep2 activity and find out potential actors of this regulation, we combined three strategies enabling the screening of suppressor mutations restoring Mep2 activity in the absence of Npr1 ( Fig. 3a and Supplementary Table 1 ). We analysed 48 suppressor mutations selected after ethyl methanesulphonate (EMS) mutagenesis conferring to Mep2 the ability to restore growth of npr1-1 cells, lacking a functional Npr1, on low ammonium medium ( Supplementary Table 1 ). We also characterized eight spontaneous suppressors obtained after prolonged incubation of npr1-1 cells on low ammonium. Finally, we screened a list of Mep2 variants described in the literature [22] , [24] , [30] or isolated in this study by site-directed mutagenesis for their ability to suppress the Npr1 requirement and confer growth, even if limited, to npr1-1 cells on low ammonium. All the isolated EMS-induced and spontaneous suppressors contained a mutation in MEP2 that turned out responsible for the suppressor phenotype. No mutation altering other proteins than Mep2, like potential partners or signalling proteins, was isolated, suggesting that the Npr1 action on Mep2 is direct. However, it cannot be excluded that Npr1 acts on Mep2 via essential or redundant proteins. The selection of such suppressors would be complicated by the reduced probability to alter an essential protein without affecting viability or to simultaneously select inactivating mutations in redundant proteins. 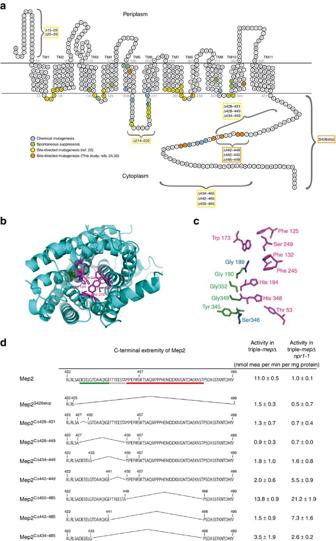Figure 3: Characterization of mutations allowing active conformations of Mep2 in the absence of a functional Npr1. (a) Topology of the Mep2 protein with the location of the mutated residues and amino-acid deletions restoring Mep2 activity in the absence of a functional Npr1. The highlighted residues correspond to the ones that were mutated by EMS mutagenesis (blue); in the spontaneous suppressors obtained on low ammonium concentrations (green); by the site-directed mutagenesis described by Van Nulandet al.22(yellow); by the site-directed mutagenesis performed in this study and by Boeckstaenset al.24,30(b,c) Location of the mutated residues close to the putative conducting pore on a model of the three-dimensional structure of Mep2, deduced from AfAmt1 crystal [PDB:2B2H17]. In magenta: residues involved in ammonium recognition and transport; in blue: mutated residues obtained by EMS mutagenesis; in green: residues mutated in spontaneous suppressors. (b) Transversal view of the Mep2 monomer, pore viewed from the extracellular side. (c) Simplified view of residues involved in ammonium recognition and transport, and mutated residues along the Mep2 pore. Lateral view, with the extracellular side above. (d) Methylammonium uptake activity of the Mep2 variants bearing truncations in the C terminus. The amino-acid sequence of the C terminus of the different Mep2 variants is represented. The sites of the truncations are indicated and S457 is labelled. The enhancer, linker and autoinhibitory domains are underlined in green, grey and red, respectively. Initial rates of [14C]-methylammonium (0.5 mM) uptake were measured from proline-grown triple-mepΔ(31019b) and triple-mepΔ npr1-1(31052c) cells transformed with YCpMep2, YCpMep2S426stop, YCpMep2CΔ442–449, YCpMep2CΔ428-449, YCpMep2CΔ434-449, YCpMep2CΔ428-431, YCpMep2CΔ434-485, YCpMep2CΔ442-485, or with YCpMep2CΔ450-485. The s.d. values are indicated for the values corresponding to the averages of two or three independent experiments. Figure 3: Characterization of mutations allowing active conformations of Mep2 in the absence of a functional Npr1. ( a ) Topology of the Mep2 protein with the location of the mutated residues and amino-acid deletions restoring Mep2 activity in the absence of a functional Npr1. The highlighted residues correspond to the ones that were mutated by EMS mutagenesis (blue); in the spontaneous suppressors obtained on low ammonium concentrations (green); by the site-directed mutagenesis described by Van Nuland et al. [22] (yellow); by the site-directed mutagenesis performed in this study and by Boeckstaens et al. [24] , [30] ( b , c ) Location of the mutated residues close to the putative conducting pore on a model of the three-dimensional structure of Mep2, deduced from AfAmt1 crystal [PDB:2B2H [17] ]. In magenta: residues involved in ammonium recognition and transport; in blue: mutated residues obtained by EMS mutagenesis; in green: residues mutated in spontaneous suppressors. ( b ) Transversal view of the Mep2 monomer, pore viewed from the extracellular side. ( c ) Simplified view of residues involved in ammonium recognition and transport, and mutated residues along the Mep2 pore. Lateral view, with the extracellular side above. ( d ) Methylammonium uptake activity of the Mep2 variants bearing truncations in the C terminus. The amino-acid sequence of the C terminus of the different Mep2 variants is represented. The sites of the truncations are indicated and S457 is labelled. The enhancer, linker and autoinhibitory domains are underlined in green, grey and red, respectively. Initial rates of [ 14 C]-methylammonium (0.5 mM) uptake were measured from proline-grown triple- mepΔ (31019b) and triple- mepΔ npr1-1 (31052c) cells transformed with YCpMep2, YCpMep2 S426stop , YCpMep2 C Δ 442–449 , YCpMep2 C Δ 428-449 , YCpMep2 C Δ 434-449 , YCpMep2 C Δ 428-431 , YCpMep2 C Δ 434-485 , YCpMep2 C Δ 442-485 , or with YCpMep2 C Δ 450-485 . The s.d. values are indicated for the values corresponding to the averages of two or three independent experiments. Full size image Overall, we characterized a collection of 70 mutated Mep2 variants able to recover activity, even if weak in some cases, in the absence of a functional Npr1 ( Fig. 3a and Supplementary Table 1 ). None of these variants recovered the major phosphorylated form in the absence of a functional kinase, consistent with Npr1 being required for Mep2 phosphorylation (data not shown). Suppressor mutations were found in all five ILs, in the cytoplasmic interfaces and in the transmembrane helices, and more particularly in TM5 and TM10, those lining the conducting pore ( Fig. 3a ). Several mutations were for instance found in physical proximity of important residues of the conducting pore, such as the gate formed by two packed phenylalanines (F132, F245) and the histidine dyad (H194, H348) proposed to play an important role in substrate translocation ( Fig. 3b,c ) [15] , [16] , [17] , [30] . Short deletions in the periplasmic N-terminal region also suppressed the Npr1 requirement, as well as the removal of G190 at the periplasmic side of TM5 ( Fig. 3a and Supplementary Table 1 ). Finally, numerous suppressor mutations were mapped in the cytosolic C terminus of Mep2. All these variants are thus able to adopt a permissive conformation allowing transport activity, circumventing the requirement of the C-terminal Npr1-dependent phosphorylation of Mep2. Together, these findings reveal a tight participation of the cytoplasmic facing domains, the ILs and the C-terminal extension in controlling Mep2 transport efficiency, and are consistent with Mep2 activity relying on an Npr1-dependent control of Mep2 conformation. The Mep2 C terminus contains distinct regulatory domains The first 22 residues of the hydrophilic C-terminal extension of Mep-Amt proteins are largely conserved and play an allosteric role in Mep-Amt activity control [31] , [32] , [33] , [34] . The conservation in the C terminus spreads beyond this domain considering several subgroups of fungal Mep-Amts ( Supplementary Fig. 5 ). Of note, 36 of 48 npr1-1 suppressors identified after EMS treatment showed mutations mapping in the third IL and in the C-terminal extension of Mep2 ( Fig. 3a and Supplementary Table 1 ). The latter were concentrated in the « YIPEPIRS » domain—residues 450–457—ending by the S457 phosphorylation site. This domain is preserved in a group of Mep2 orthologues, including CaMep2 from the human pathogen Candida albicans ( Supplementary Fig. 5 ). Mutations of the proline residues (P452, P454) in this domain were found as alleviating the Npr1 requirement to Mep2 activity ( Supplementary Table 1 ), suggesting that an alteration of the local structure could prevent the negative regulation of transport by the C-terminal extension. Deletion of the C terminus of a bacterial and a fungal Mep-Amt protein has been shown to strongly reduce, but not completely turn off, transport [34] , [35] , [36] . A Mep2 version lacking the complete C terminus (Mep2 S426stop ), that we defined as the ‘hydrophobic core’ of Mep2, also displayed a reduced transport activity ( Fig. 3d ). Consistently, the truncated protein Mep2 S426stop shows a fourfold lower V max for [ 14 C]-methylammonium (4.23±0.45 nmol min −1 per mg protein.) compared with native Mep2 (17.5 nmol min −1 per mg protein [25] ) and a nearly sixfold lower affinity (Mep2: 0.34 mM (ref. 25 ); Mep2 S426stop : 1.95±0.01 mM). Nevertheless, the residual activity of Mep2 S426stop was able to slightly repair the growth defect of triple- mepΔ cells on low ammonium, and this phenotype was not altered in the absence of Npr1 ( Supplementary Fig. 6 ). Hence, the Mep2 hydrophobic core possesses a basal transport activity but the C terminus plays a significant role in the optimal transport function of Mep2. The Mep2 C terminus appears additionally required for the Npr1-mediated regulation of transport activity in keeping with the role of S457 phosphorylation. We next focused on measuring the activity of Mep2 proteins bearing internal truncations in the C terminus. From the results of activity measurements ( Fig. 3d ) and growth tests (data not shown), three domains in the Mep2 C terminus were revealed as being involved in activity tuning. Mep2 versions bearing deletions before F442 are inactive regardless of Npr1 integrity. An enhancer domain, required for optimal Mep2 activity independently of Npr1 regulation, is limited to residues 428–441 and is comprised in the region of the Mep2 C terminus conserved in the Mep-Amt family. The enhancer domain sticks to what we define as a linker domain limited to residues 442–449. The linker domain is still required for optimal Mep2 activity in the presence of Npr1 but dispensable when the kinase integrity is altered. The linker domain is followed by an area of negative regulation between residues 450 and 485, comprising the ‘YIPEPIRS’ stretch and thus S457, and the above-mentioned prolines. This negative domain is dispensable for Mep2 activity in the presence as in the absence of Npr1 and is thus required for the autoinhibition of Mep2 occurring upon the loss of kinase integrity. A Mep2 variant lacking this domain is thus active, and even hyperactive, in Npr1-lacking cells. These data indicate that in the presence of Npr1, the autoinhibitory domain is maintained silent whereas the enhancer domain is free to activate the hydrophobic core of Mep2. Npr1 thus exerts a positive control on Mep2 activity by preventing the autoinhibitory domain to counteract activation of the hydrophobic core by the enhancer domain. Hence, in native Mep2, phosphorylation at S457 is not directly required for Mep2 activity but rather inhibits the autoinhibitory C-terminal domain. Overall, the two phosphorylated Mep2 forms correspond to conformational states controlled by a specific interplay of separated C-terminal domains. Our data are consistent with a particular spatial organization of the different domains of the C terminus being responsible for the control of Mep2 activity. Glutamine triggers TORC1-dependent inactivation of Mep2 We next addressed the physiological parameters tuning the Mep2 activity via Npr1. Glutamine is a preferred nitrogen source known to modify the phosphorylation state of Npr1 and assumed to inactivate the kinase through a TORC1-dependent mechanism [4] , [6] . We tested the effect of glutamine addition on the ability of Mep2 to transport ammonium and on the electrophoretic profile of the transport protein. Glutamine addition to cells growing under poor nitrogen supply triggered a rapid arrest in the Mep2-mediated ammonium removal from the medium ( Fig. 4a ) and an instant dephosphorylation of Mep2 N4Q ( Fig. 4b,c ), without altering cell surface localization of the transport protein ( Supplementary Fig. 7 ). Hence, as for Npr1 inactivation, glutamine supplementation triggers Mep2 inactivation and a quick loss of the S457-phosphorylated Mep2 form ( Fig. 4c ). Furthermore, addition of rapamycin to cells growing under poor nitrogen supply to hinder TORC1 activity prior to glutamine addition protected Mep2 against loss of the phosphorylated form ( Fig. 4d ). The glutamine effect on Mep2 regulation is thus largely dependent on the TORC1 pathway. Of note, addition of rapamycin alone to cells growing under poor nitrogen supply increased the proportion of the S457-phosphorylated Mep2 form, consistent with downregulation of TORC1 activity in these conditions stimulating Mep2 phosphorylation ( Fig. 4d ). Glutamine addition induced phosphorylation of Npr1, a process that was inhibited by former incubation of the cells with rapamycin ( Fig. 4d ). Hence, TORC1 triggers the phosphorylation of the kinase upon transferring the cells to a preferred nitrogen supplementation, in keeping with previous data [3] , [37] . Rapamycin addition had no major impact on the cell surface localization of Mep2 ( Supplementary Fig. 7 ). 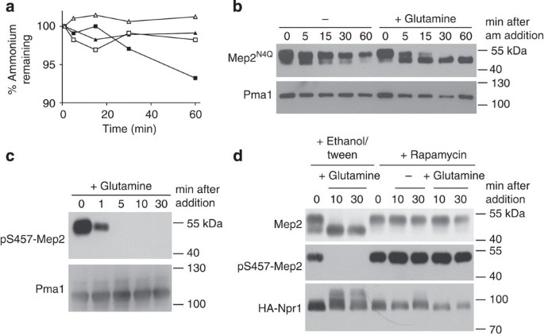Figure 4: Glutamine triggers TORC1-dependent inactivation of Mep2. (a) Triple-mepΔ(31019b, black symbols) and triple-mepΔ npr1-1(31052c, white symbols) cells transformed with YCpMep2N4Qwere grown in the presence of proline (0.1%). At timet=0, ammonium (2 mM) with (triangles) or without (squares) glutamine (gln, 0.1%) was added to the cell cultures of identical optical density. Ammonium remaining in the medium, expressed as percentage of the initial concentration, was monitored for 1 h. (b,c) Membrane-enriched extracts were prepared from proline-grown triple-mepΔ(31019b) cells transformed with YCpMep2N4Q. (b) Immunodetection of Mep2N4Qand Pma1 (loading control). At timet=0, ammonium (2 mM) with or without (−) glutamine (0.1%) was added to the cell culture. (c) Immunodetection of pS457-Mep2 and Pma1 (loading control). At timet=0, glutamine (0.1%) was added to the cell culture. (d) Immunodetection of Mep2 and pS457-Mep2 from membrane-enriched extracts treated with N-glycosidase F of proline-grown wild-type (23344c) cells. Immunodetection of HA-Npr1 from total extracts of proline-grownnpr1Δ(30788a) cells transformed with pAS103 (YEpHA-Npr1). At timet=0, rapamycin (2 μg ml−1) or the rapamycin vehicle alone (control, ethanol/tween) was added to the cell culture. 1 h later (t0), glutamine (0.1%) was added or not (−) to the cell culture. Figure 4: Glutamine triggers TORC1-dependent inactivation of Mep2. ( a ) Triple- mepΔ (31019b, black symbols) and triple- mepΔ npr1-1 (31052c, white symbols) cells transformed with YCpMep2 N4Q were grown in the presence of proline (0.1%). At time t =0, ammonium (2 mM) with (triangles) or without (squares) glutamine (gln, 0.1%) was added to the cell cultures of identical optical density. Ammonium remaining in the medium, expressed as percentage of the initial concentration, was monitored for 1 h. ( b , c ) Membrane-enriched extracts were prepared from proline-grown triple- mepΔ (31019b) cells transformed with YCpMep2 N4Q . ( b ) Immunodetection of Mep2 N4Q and Pma1 (loading control). At time t =0, ammonium (2 mM) with or without (−) glutamine (0.1%) was added to the cell culture. ( c ) Immunodetection of pS457-Mep2 and Pma1 (loading control). At time t =0, glutamine (0.1%) was added to the cell culture. ( d ) Immunodetection of Mep2 and pS457-Mep2 from membrane-enriched extracts treated with N-glycosidase F of proline-grown wild-type (23344c) cells. Immunodetection of HA-Npr1 from total extracts of proline-grown npr1Δ (30788a) cells transformed with pAS103 (YEpHA-Npr1). At time t =0, rapamycin (2 μg ml −1 ) or the rapamycin vehicle alone (control, ethanol/tween) was added to the cell culture. 1 h later (t0), glutamine (0.1%) was added or not (−) to the cell culture. Full size image The phosphorylation status and activity of the Npr1 kinase are assumed to be controlled by TORC1 via the Sit4 phosphatase [38] . SIT4 deletion is accompanied by Npr1 hyperphosphorylation and likely inactivation [39] . We likewise observed hyperphosphorylation of Npr1 in the absence of Sit4 ( Supplementary Fig. 8a ). However, SIT4 deletion did not mimic the absence of Npr1, as Mep2 was still detected as two forms in a sit4Δ mutant, like in wild-type cells ( Supplementary Fig. 8b ). Measurement of [ 14 C]-methylammonium accumulation further sustains that the ammonium transport proteins are still active in the absence of Sit4 ( Supplementary Fig. 8c ) [3] . Hence, in the tested conditions, the Npr1 activity required for the Mep2 control appears conserved in the absence of Sit4, even though the kinase is hyperphosphorylated. We further observed a synthetic lethality upon combining NPR1 and SIT4 gene deletions. Our data on the Mep2 control indicate that Npr1 and Sit4 can also act in independent pathways. Although the Mep2 regulation by Npr1 does not involve endocytosis and destabilization of the transport system, we reasoned that arrestin-like proteins might nevertheless act as adaptors of other regulatory factors than ubiquitin ligases, involved in the Mep2 inactivation process. Deletion of all 10 arrestin-like proteins identified in yeast did, however, not protect from the loss of the Mep2 phosphorylated form occurring upon glutamine addition ( Supplementary Fig. 9 ). Hence, the inherent activity control of Mep2 mediated by glutamine is independent of these arrestin-like adaptors. Plasma membrane Psr1 and Psr2 mediate Mep2 dephosphorylation Our data are consistent with Mep2 being inactivated upon dephosphorylation of S457, as occurs upon glutamine supplementation. To identify the phosphatase(s) involved in Mep2 dephosphorylation, we screened a library of 30 strains, each bearing the deletion of one of each non-essential serine/threonine phosphatase gene ( Supplementary Table 2 ). Mep2 was immunodetected from protein extracts from mutant cells growing on proline medium and after 30 min of glutamine supplementation. When a protection against Mep2 dephosphorylation was observed with a strain, even partial, the phenotype was retested after deletion of the concerned phosphatase gene in an independent Σ1278b laboratory background. We found that the single deletion of the PSR1 and PSR2 phosphatase genes partially protected Mep2 from glutamine-induced dephosphorylation, suggesting a redundant function of both Psr proteins ( Fig. 5a ). Consistently, double psr1Δ psr2Δ -mutant cells were fully protected against glutamine-induced S457 dephosphorylation of Mep2. Psr1 and Psr2 are two plasma membrane phosphatases so far mainly described for their role in sodium resistance and Msn2/4 activation [40] , [41] . Our data reveal Psr1 and Psr2 as two redundant phosphatases required for glutamine-induced Mep2 dephosphorylation. 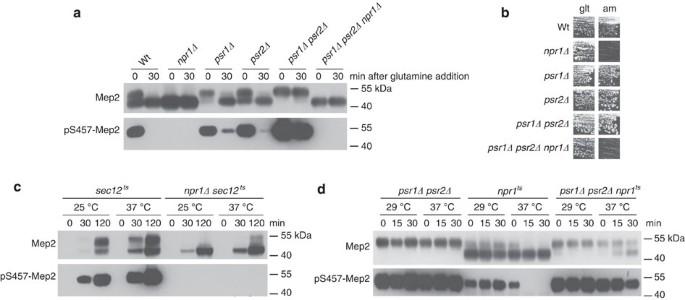Figure 5: Plasma membrane Psr1 and Psr2 mediate Mep2 dephosphorylation. (a,b) Wild-type (Wt, 23344c),npr1Δ(30788a),psr1Δ(PVV62),psr2Δ(PVV68),psr1Δ psr2Δ(PVV110) andpsr1Δ psr2Δ npr1Δ(PVV115) cells were used. (a) Immunodetection of Mep2 and pS457-Mep2 from membrane-enriched and glycosidase-treated extracts of proline-grown cells. (b) Growth tests on solid medium containing, as the sole nitrogen source, 3 mM ammonium (am) or 0.1% glutamate (glt, positive growth control). Cells were incubated at 29 °C for 3 days. (c) Immunodetection of neosynthesized Mep2 and pS457-Mep2 from membrane-enriched cell extracts treated withN-glycosidase F. Mep2 neosynthesis was induced by transferringsec12ts(NY738) andsec12tsnpr1Δ(MB262) cells from a nitrogenous-repressive medium (glutamine 0.1% and ammonium 100 mM) to a derepression medium (proline 0.1%), at the permissive (25 °C) and restrictive (37 °C) temperatures. (d) Immunodetection of Mep2 and pS457-Mep2 from membrane-enriched cell extracts treated withN-glycosidase F.psr1Δ psr2Δ(PVV110),npr1ts(33035b) andpsr1Δ psr2Δ npr1ts(36323c) cells were grown at the permissive temperature (29 °C) in the presence of proline (0.1%). At time 0, cells were transferred in a similar proline medium preheated at the permissive (29 °C) or restrictive (37 °C) temperatures. Figure 5: Plasma membrane Psr1 and Psr2 mediate Mep2 dephosphorylation. ( a , b ) Wild-type (Wt, 23344c), npr1Δ (30788a), psr1Δ (PVV62), psr2Δ (PVV68), psr1Δ psr2Δ (PVV110) and psr1Δ psr2Δ npr1Δ (PVV115) cells were used. ( a ) Immunodetection of Mep2 and pS457-Mep2 from membrane-enriched and glycosidase-treated extracts of proline-grown cells. ( b ) Growth tests on solid medium containing, as the sole nitrogen source, 3 mM ammonium (am) or 0.1% glutamate (glt, positive growth control). Cells were incubated at 29 °C for 3 days. ( c ) Immunodetection of neosynthesized Mep2 and pS457-Mep2 from membrane-enriched cell extracts treated with N -glycosidase F. Mep2 neosynthesis was induced by transferring sec12 ts (NY738) and sec12 ts npr1Δ (MB262) cells from a nitrogenous-repressive medium (glutamine 0.1% and ammonium 100 mM) to a derepression medium (proline 0.1%), at the permissive (25 °C) and restrictive (37 °C) temperatures. ( d ) Immunodetection of Mep2 and pS457-Mep2 from membrane-enriched cell extracts treated with N -glycosidase F. psr1Δ psr2Δ (PVV110), npr1 ts (33035b) and psr1Δ psr2Δ npr1 ts (36323c) cells were grown at the permissive temperature (29 °C) in the presence of proline (0.1%). At time 0, cells were transferred in a similar proline medium preheated at the permissive (29 °C) or restrictive (37 °C) temperatures. Full size image To date, Npr1 is reported to regulate the stability of amino-acid transporters by controlling the phosphorylation state of arrestin-like intermediate proteins [2] , [3] . The rapid Npr1-dependent dephosphorylation of Mep2 at the plasma membrane suggests that Npr1 could regulate the activity of the redundant phosphatases. To test whether Npr1 controls the Mep2 phosphorylation status by inhibiting the Psr phosphatases, we assessed Mep2 phosphorylation in triple psr1Δ psr2Δ npr1Δ -mutant cells. In these cells, Mep2 was immunodetected as a dephosphorylated form, lacking phosphorylation at S457 ( Fig. 5a ). Consistently, growth of psr1Δ psr2Δ npr1Δ cells was affected on low ammonium, similarly to npr1Δ cells ( Fig. 5b ). Npr1 is thus directly or indirectly involved in the phosphorylation step of Mep2. We next used a thermosensitive sec12 ts mutant, affected in vesicles exit from the endoplasmic reticulum (ER) [42] to test whether Mep2 can be phosphorylated in the ER. We first ascertained that, at 25 °C, neosynthesized Mep2 reaches the plasma membrane of these cells, whereas the transport protein is blocked in the internal membranes, the perinuclear and peripheral ER, at 37 °C ( Supplementary Fig. 10 ). At this restrictive temperature, neosynthesized Mep2 was immunodetected as two major bands in the sec12 ts mutant ( Fig. 5c ). The Mep2 upper form was also immunodetected with the pS457 antibodies showing that the major phosphorylation of Mep2 can occur when the protein is trapped in the ER. Mep2 neosynthesized in sec12 ts npr1Δ double mutant cells at 37 °C appeared as a major band with an upper faint smear that did not cross-react with the pS457 antibodies ( Fig. 5c ). The Npr1 kinase is thus either directly or indirectly required for the S457 phosphorylation step of Mep2, as the transport protein is synthesized in the ER. We next assessed whether Mep2 dephosphorylation occurring upon Npr1 inactivation requires the Psr phosphatases. We used a psr1Δ psr2Δ npr1 ts mutant allowing Mep2 phosphorylation at the permissive temperature and checked the fate of S457 phosphorylation upon thermosensitive inactivation of Npr1 ( Fig. 5d ). S457 phosphorylation of Mep2 was rapidly lost when npr1 ts cells were shifted at 37 °C, whereas it was largely preserved in psr1Δ psr2Δ npr1 ts cells indicating that S457 dephosphorylation upon Npr1 inactivation requires the Psr phosphatases. Hence, the Mep2 phosphorylation status appears controlled by a dynamic process implying a balance between Npr1-dependent phosphorylation and Psr-dependent dephosphorylation of Mep2, involving a role of Npr1 at the birth of Mep2 in the ER and at the plasma membrane. Mep2 activity requires the TORC1 upstream regulator Npr2 Yeast Npr2 belongs to a family of conserved proteins of unknown function; its human orthologue, NPRL2, being recognized as a tumour suppressor [43] , [44] . As NPRL2, yeast Npr2 belongs to a recently identified GTPase activating complex, transmitting an amino-acid deprivation signal to TORC1 (refs 45 , 46 ). Npr2-lacking cells are reported to be affected for growth on ammonium but the underlying mechanism is unknown [7] , [44] . Cells expressing Mep2 as sole Mep-Amt protein and lacking Npr2 displayed strongly altered growth in the presence of low ammonium ( Fig. 6a ). In Npr2-lacking cells, Mep2 was detected as one major form, lacking S457 phosphorylation, like in the absence of Npr1 ( Fig. 6b ). Hence, Npr2 is required for S457 phosphorylation and for Mep2 function. Npr1 is reported to be hyperphosphorylated in the absence of Npr2 (ref. 7) [7] . Here, we show that expression of HA-Npr1 from an episomal plasmid in Npr2-lacking cells restored growth on ammonium ( Supplementary Fig. 11 ) and S457 phosphorylation of Mep2 ( Fig. 6c ). Hence, NPR1 overexpression suppresses the deleterious effect of NPR2 deletion on Mep2 activity and phosphorylation status. 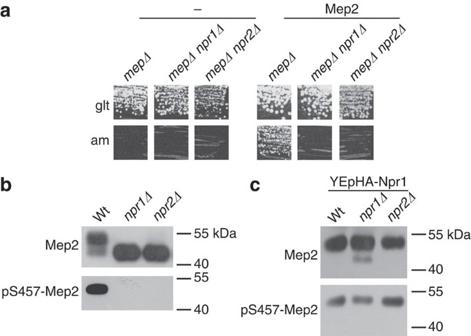Figure 6: Mep2 activity requires the TORC1 upstream regulator Npr2. (a) Growth tests on solid medium containing, as the sole nitrogen source, 3 mM ammonium (am) or 0.1% glutamate (glt, positive growth control). Triple-mepΔ(31019b), triple-mepΔ npr1-1(31052c) and triple-mepΔ npr2Δ(FV389) cells transformed with pFL38 (−) or YCpMep2 (Mep2) were incubated for 3 days at 29 °C. (b,c) Immunodetection of Mep2 and pS457-Mep2 from membrane-enriched and glycosidase-treated extracts. Wild type (Wt, 23344c),npr1Δ(30788a) andnpr2Δ(FV388) were grown with proline (0.1%) as nitrogen source. (c) Cells were transformed with pAS103 (YEpHA-Npr1). Figure 6: Mep2 activity requires the TORC1 upstream regulator Npr2. ( a ) Growth tests on solid medium containing, as the sole nitrogen source, 3 mM ammonium (am) or 0.1% glutamate (glt, positive growth control). Triple- mepΔ (31019b), triple- mepΔ npr1-1 (31052c) and triple- mepΔ npr2Δ (FV389) cells transformed with pFL38 (−) or YCpMep2 (Mep2) were incubated for 3 days at 29 °C. ( b , c ) Immunodetection of Mep2 and pS457-Mep2 from membrane-enriched and glycosidase-treated extracts. Wild type (Wt, 23344c), npr1Δ (30788a) and npr2Δ (FV388) were grown with proline (0.1%) as nitrogen source. ( c ) Cells were transformed with pAS103 (YEpHA-Npr1). Full size image Npr2, the upstream regulator of TORC1, thus controls Mep2 phosphorylation and activity via the effector kinase Npr1. This study reports that the TORC1 effector kinase Npr1 regulates the inherent activity of the plasma membrane Mep2 ammonium transport protein. We show that Npr1 is not required for synthesis, plasma membrane targeting and stability of Mep2. Npr1 instead exerts a positive control on Mep2 by mediating S457 phosphorylation, which in turn silences a C-terminal autoinhibitory domain of the transport protein. Hence, in addition to its role in arrestin-mediated endocytosis of transporters [2] , [3] , Npr1 also tunes nutrient permeability. Amino-acid availability is one of the nutrient signals integrated by TORC1 to control cell growth. Glutamine is a particular amino acid, playing a central role in nitrogen metabolism in general as it is, with glutamate, the main nitrogen donor for the biosynthesis of nitrogen-containing compounds such as other amino acids and nucleotides. In yeast, sufficient glutamine supply further promotes nitrogen catabolite repression, regulating the transcription of genes to favour preferred nitrogen sources utilization [47] . Addition of the preferred glutamine nitrogen source to cells growing under poor nitrogen supply also triggers TORC1-dependent phosphorylation and likely inactivation of Npr1 (refs 4 , 6 ). We show that Npr1 inactivation, upon glutamine supplementation or as artificially induced by use of a thermosensitive Npr1 variant, correlates with instant S457 dephosphorylation and rapid inactivation of plasma membrane Mep2. Furthermore, we identify plasma membrane Psr1 and Psr2 as redundant phosphatases required for the Mep2 dephosphorylation. These data reveal a new role for the Psr proteins in the regulation of ammonium transport in addition to their role in sodium and stress response [40] , [41] . TORC1 is reported to inactivate Npr1 via inhibition of the Sit4 phosphatase [38] . However, Sit4 seems not involved in the Mep2 activity regulation. Interestingly, despite its hyperphosphorylated state in the absence of Sit4, Npr1 apparently conserves activity, at least in Mep2 phosphorylation. Sit4 and Npr1 could also act in parallel pathways as supported by the synthetic lethality. Overall, the correlation between hyperphosphorylation of Npr1 and inactivation of the kinase is not so straightforward. Particular Npr1 phosphorylation sites are likely involved in the kinase activity regulation. Our data are consistent with TORC1-mediating Npr1 phosphorylation upon preferred nitrogen source supplementation, in keeping with previous observations [3] , [4] . This study also reveals Npr2 as an upstream regulator of the Mep2 control. How the amino-acid signal is transmitted to TORC1 is not fully understood. In both mammalian and yeast cells, TORC1 localizes at the lysosomal/vacuolar membrane [48] . Npr2 was recently shown to belong to a conserved GTPase activating complex, GATOR1, also located at the lysosomal/vacuolar membrane and mediating an amino-acid deprivation signal to TORC1 (refs 45 , 46 , 49 ). Interestingly, Npr1 binds to several components of the TORC1 complex [37] and rapamycin treatment induces the recruitment of a fraction of Npr1 to the plasma membrane [2] . Plasma membrane docking of released Npr1 likely favours interaction and phosphoinhibition of arrestin-like proteins, as shown for Art1, preventing endocytosis of transporters. This docking could also favour direct phosphorylation and activity of plasma membrane Mep2. Npr1-dependent phosphorylation would additionally target Mep2 in internal membranes as shown here for nascent Mep2 in the ER. Together, our data indicate that Npr1 and the Psr phosphatases control a dynamic process of Mep2 activation/inactivation by phosphorylation/dephosphorylation, the balance being tuned via the TORC1 pathway according to the quality of the nitrogen supply ( Fig. 7a ). 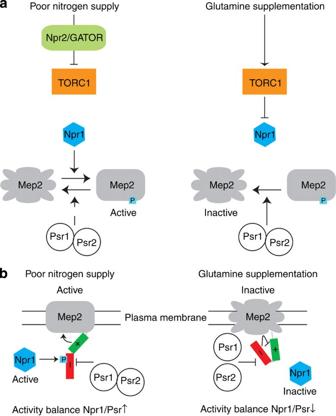Figure 7: Model of Mep2 regulation by the TORC1 effector kinase Npr1. (a) Left panel: During poor nitrogen supply, TORC1 activity is decreased via the GATOR1 complex including the Npr2 protein. Npr1 is active and enables S457 phosphorylation and activity of Mep2. Right panel: Upon glutamine supplementation, TORC1 is upregulated and Npr1 is downregulated. The Psr1 and Psr2 phosphatases enable dephosphorylation and thus inactivation of Mep2. This model does not discard an additional control of the activity of the Psr phosphatases by TORC1/Npr1 or other pathways. (b) Left panel: In the presence of poor nitrogen supply, the Npr1 kinase is active and enables S457 phosphorylation and silencing of the C-terminal autoinhibitory domain of Mep2. The enhancer C-terminal domain of Mep2 is free to activate the transport protein. The Psr1 and Psr2 phosphatases are also, at least partially, active in these conditions and mediate Mep2 dephosphorylation. Phosphorylated and non-phosphorylated Mep2 coexist in these conditions. Right panel: Upon glutamine supplementation, the Npr1 control is relieved and plasma-membrane Mep2 are rapidly dephosphorylated via the Psr phosphatases. The non-phosphorylated autoinhibitory domain of Mep2 prevents the enhancer domain to activate the transport protein. Figure 7: Model of Mep2 regulation by the TORC1 effector kinase Npr1. ( a ) Left panel: During poor nitrogen supply, TORC1 activity is decreased via the GATOR1 complex including the Npr2 protein. Npr1 is active and enables S457 phosphorylation and activity of Mep2. Right panel: Upon glutamine supplementation, TORC1 is upregulated and Npr1 is downregulated. The Psr1 and Psr2 phosphatases enable dephosphorylation and thus inactivation of Mep2. This model does not discard an additional control of the activity of the Psr phosphatases by TORC1/Npr1 or other pathways. ( b ) Left panel: In the presence of poor nitrogen supply, the Npr1 kinase is active and enables S457 phosphorylation and silencing of the C-terminal autoinhibitory domain of Mep2. The enhancer C-terminal domain of Mep2 is free to activate the transport protein. The Psr1 and Psr2 phosphatases are also, at least partially, active in these conditions and mediate Mep2 dephosphorylation. Phosphorylated and non-phosphorylated Mep2 coexist in these conditions. Right panel: Upon glutamine supplementation, the Npr1 control is relieved and plasma-membrane Mep2 are rapidly dephosphorylated via the Psr phosphatases. The non-phosphorylated autoinhibitory domain of Mep2 prevents the enhancer domain to activate the transport protein. Full size image This study also provides evidence for the molecular mechanism of Npr1-mediated regulation of Mep2. Structural data of bacterial Mep-Amt trimers indicate that the conserved domain of the C terminus of one monomer interacts with ILs of its own subunit and with the loops of the contiguous one [17] , [50] . The conserved portion of the C-terminal domain of Mep-Amt proteins is further reported to trans-activate the monomers via an allosteric switch [32] , [33] , [34] . Here, we show that the Mep2 C terminus contains at least three functional domains. The conserved enhancer domain improves the basal activity of the lone hydrophobic core of Mep2 and is connected by a linker domain to an autoinhibitory domain comprising S457 and mediating the transport activity control by Npr1. The kinase thus positively controls Mep2 activity via a phosphoinhibition maintaining the autoinhibitory domain silent and unable to counteract activation of the hydrophobic core by the enhancer domain ( Fig. 7b ). Npr1 is thus required to keep Mep2 in an active conformation. Numerous npr1 suppressors in Mep2 lie in the TM5 and TM10 domains longing the conducting pore, in the IL3 linking TM5 and TM6, and in a segment of the autoinhibitory C-terminal domain. Interactions between IL3 and the C-terminal extremity might control the conformation of the conducting pore and thereby the fine tuning of Mep2 activity by governing the inclination of TM5, as proposed for Escherichia coli AmtB [51] . In the latter, like in most bacterial Mep-Amts, the C terminus stops after the conserved domain. Negative regulation of AmtB activity is achieved by the binding to the C terminus of the GlnK partner that blocks the cytoplasmic exit of the conducting pore [50] , [52] . Yet, GlnK is only found in bacteria and a few plant species. The potential role of the extended and variable C-terminal tail found in most eukaryotic Mep-Amt-Rh proteins is largely unknown. The autoinhibitory role of the Mep2 C-terminal extension apparently contrasts with the situation of AtAmt1;1, in Arabidopsis thaliana , where transport inactivation is rather correlated to a phosphorylation in the conserved domain, corresponding to the activating region [53] . There are obviously different ways to alter the spatial organization and interaction of the C terminus with the conducting hydrophobic core of Mep-Amts to control their activity. A similar mechanism of activity fine tuning involving the C terminus might also apply to mammalian Rh factors, despite the divergence of this domain. We recently characterized a human polymorphism of RhCG showing a reduced activity and likely affected in the interaction between IL3 and the C terminus [54] . The clinical outcome potentially associated to this variant is currently unknown. We expect that the TORC1-Npr1 control of transport activity will target other proteins than Mep2. For instance, the Mep1 and Mep3 ammonium transport proteins also appear regulated by Npr1 at the level of their inherent activity (Boeckstaens and colleagues, in preparation) [23] , [24] . A sustained negative regulation of Mep2 activity by glutamine might reflect a hierarchy in the utilization of preferred nitrogen sources. A mechanism of Mep2 fine tuning and shut-off in the presence of sufficient glutamine might further participate to the control of the dimorphic change leading to filamentation. Indeed, the Mep2 transport efficiency and its capacity to allow filamentation are tightly linked [24] , [55] . We anticipate that yeast cells have evolved a mechanism finely controlling the plasma membrane permeability with an ordered selection of transport proteins to be inactivated but preserved at the plasma membrane for possible reactivation, endocytosed or maintained active. This strategy could enable a fast and flexible adaptation to face environmental perturbation of nutrient availability. Our study thus adds to the roles of TORC1 in the control of transcription, translation, autophagy and endocytosis, a role in the tuning of plasma membrane uptake activity. An involvement of the conserved mTORC1 pathway in the control of inherent activity of transport proteins remains to be evaluated in the mammalian context. Strains and growth conditions The S. cerevisiae strains used in this study are listed in Supplementary Table 3 . Part of these strains are isogenic with the wild-type Σ1278b [56] . Strains BY4741, BY4742, NY13, TB50 and those deriving from them are isogenic with S288c. Cells were transformed by heat shock (42 °C) after permeabilization with lithium acetate (100 mM) treatment [57] . Gene deletions were performed by homologous recombination, replacing the gene to delete by a kanMX or hphMX cassette conferring resistance to geneticin or hygromycin B to the cells, respectively [58] . Cells were grown in a minimal buffered (pH 6.1) medium with 3% glucose as the carbon source [59] . In experiments in which genes were expressed under the GAL1 promoter, 3% galactose+0.3% glucose were used for transcriptional induction, and 3% glucose for repression. To this medium, nitrogen sources were added as required by the experiment and as specified in the text. The nitrogen sources used were 0.1% proline, 0.1% glutamine, 0.1% glutamate or (NH 4 ) 2 SO 4 at the specified concentration. When required, the medium was supplemented with 0.0025% uracil, histidine, methionine, tryptophane or/and 0.005% leucine to complement auxotrophies. Rapamycin (LC Laboratories) was used at a final concentration of 2 μg ml −1 from a stock solution prepared in 90% ethanol/10% Tween-20. Plasmids and mutagenesis Plasmids used in this study are listed in Supplementary Table 4 . Primers used in this study are listed in Supplementary Table 5 . Site-directed mutagenesis of MEP2 were performed using the Quick Change Site-directed Mutagenesis Kit (Stratagene). Correct mutagenesis was checked by sequencing. pGAL1Mep2-GFP: the required MEP2 fragments were amplified by PCR using YCpMep2 vector [11] as template and then cloned by yeast in vivo recombination in the pGAL1Gap1-GFP vector [5] . pGAL1Mep2 N4Q -GFP and YCpMep2 S426stop : the required MEP2 fragments were amplified using the YCpMep2 N4Q vector [25] and the YCpMep2 vector [11] , respectively, and similarly cloned in pGAL1Mep2-GFP and YCpMep2, respectively. YCpMep2-GFP: the required MEP2 fragments were amplified by PCR using pGALMep2-GFP vector as template and then cloned by yeast in vivo recombination in the YCpMep2 vector [11] . Spontaneous suppressors mep1Δ mep3Δ npr1-1 (31059d) cells transformed with pGAL1MEP2 N4Q -GFP were spread on a minimal medium containing 1 mM ammonium as nitrogen source and incubated at 29 °C for more than 2 weeks. EMS mutagenesis Ethyl methanesulphonate (EMS) mutagenesis [60] was performed on triple- mepΔ npr1-1 (31052c) cells transformed with pGAL1-MEP2 N4Q -GFP. Cells were resuspended in a phosphate buffer pH8 containing 2% glucose and then incubated at 30 °C during 30, 50 or 70 min in the presence of EMS. Mutagenesis was stopped by the addition of an equal volume Na 2 S 2 O 3 and cells were spread on a selection medium containing galactose (3%) and glucose (0.3%) as carbon sources and ammonium (3 mM) as nitrogen source. Western immunoblotting For total protein extracts, about 5.10 7 yeast cells were filtered (Millipore 0.45 μm), lysed in the presence of NaOH (0.2 M) and the proteins were precipitated by trichloroacetic acid (TCA, 5%) addition. The precipitates were neutralized and dissolved in 50 μl of a V/V 1 M Tris base/sample buffer (100 mM Tris-HCl, pH 6.8, 4 mM EDTA, 4% SDS, 20% glycerol, 0.02% bromophenol blue) containing 2% 2-mercaptoethanol and heated for 10 min at 37 °C (membrane proteins) or 95 °C (soluble proteins). For membrane-enriched preparations, about 10 8 yeast cells were filtered (Millipore 0.45 μm), washed with cold water, and resuspended in 0.2 ml lysis buffer (0.1 M Tris-HCl pH 7.5; 0.15 M NaCl; 5 mM EDTA) containing proteinase inhibitors (Complete Mini, Roche). An equal volume of glass beads was added and cells were lysed at 4 °C in a 2.0 ml Eppendorf tube by vortex mixing for 2 min. The extracts were diluted with 2 volumes of lysis buffer and centrifuged for 5 min at 3,000 r.p.m. to remove unbroken cells and large debris. The plasma membrane-enriched fraction was collected by centrifugation for 45 min at 12,000 r.p.m. For blot analysis, equal protein amounts (~20 μg) were loaded onto a 6 to 8% SDS–polyacrylamide gel in a Tricine system [61] . After transfer to a nitrocellulose membrane (Protran, VWR), proteins were probed with a mouse or rabbit antiserum raised against the C-terminal region of Mep2 (1:2,000) [25] , a peptide (PEPIRpSKTSAQM) centred on phosphoS457 of Mep2 (Genecust), HA (1:10,000) (Roche, 11666606001), GFP (1:10,000) (Roche, 11814460001) and Pma1 (1:10,000) [5] . Primary antibodies were detected with horseradish-peroxidase-conjugated anti-rabbit- or anti-mouse-IgG secondary antibodies (GE Healthcare, NA931 and NA934, respectively) followed by measurement of chemiluminescence (Lumi-Light PLUS , Roche). Uncropped scans of the most important western blots were supplied as Supplementary Fig. 12 . For ALP treatment on membrane-enriched cell extracts, the collected membrane pellet was suspended in phosphatase buffer CIP 1 × added of 0.1% SDS, 2 mM PMSF and proteinase inhibitors (Complete Mini, Roche). The extracts were then incubated 1 h at 37 °C in the presence (or not) of 10 units of calf ALP (Roche). Proteins were precipitated with 10% TCA. For λ phosphatase treatment on membrane-enriched cell extracts, the collected membrane pellet was suspended in 1 × NEBuffer for Protein MetalloPhosphatases (50 mM HEPES, 100 mM NaCl, 2 mM DTT, 0.01% Brij 35, pH 7.5; New England BioLabs) supplemented with 1 mM MnCl 2 , 0,25 mg ml −1 Triton X-100 and proteinase inhibitors (Complete Mini, Roche). The extracts were then incubated 1 h at 30 °C in the presence (or not) of 40 units of Lambda Protein Phosphatase (New England BioLabs). Proteins were precipitated with 10% TCA. For PNGase F treatment on membrane-enriched cell extracts, the collected membrane pellet was suspended in buffer (1 × PBS, 10 mM EDTA pH8, 0.5% octyl glucopyranoside, 0.2% 2-mercaptoethanol, 3 mM PMSF and proteinase inhibitors) and incubated 1 h at 37 °C in the presence (or not) of 1 unit of peptide- N -glycosidase F (PNGase F, Roche). Proteolytic shaving About 5.10 8 yeast cells were collected and resuspended in 1 ml spheroplasting buffer (1 M sorbitol, 0.1 mM EDTA pH 7.5, 0.5% 2-mercaptoethanol). Protoplasts were prepared by incubating the cells for 20 min at 30 °C in the presence of 20 U ml −1 lyticase (Roche). Intact protoplasts were then collected by centrifugation at 4,000 g for 2 min and the pellet was resuspended in 100 μl spheroplasting buffer. The protoplasts were digested for 15 min at 25 °C in the presence of proteinase K (Roche; 0, 10 or 50 μg) or trypsin (Sigma; 0, 50 or 200 μg). Proteins were precipitated with TCA. [ 14 C]-methylammonium uptake assays Initial rates of [ 14 C]-methylammonium (BioActif) uptake were measured as described for amino acids with cells grown in minimal medium containing proline as nitrogen source. Briefly, 5-ml samples of an exponentially growing culture corresponding to about 0.25 mg protein per ml were put, without any change of the medium, into vessels containing the labelled methylammonium and preheated to 29 °C or 37 °C in a rotary water bath. One-millilitre samples were then removed at time intervals and poured onto filters (0.45 μM, Millipore), which were immediately washed five times with 2 ml iced water before counting. Ammonium removal assays At time t =0, ammonium (2 mM) was added to the cell culture together with glutamine (0.1%) or not. Samples of medium supernatant were withdrawn at time intervals and assayed for ammonium concentration by enzymatic coupling with L -glutamate dehydrogenase (Roche) [62] . Fluorescence microscopy Cells were viewed with a Nikon Eclipse E600 microscope equipped with fluorescence light filter sets (450–490 nm). Images were captured with a Nikon DXM1200 digital camera and processed with Adobe Photoshop 5.0 (Adobe Systems, Mountain View, CA). Computer analysis Mep2 protein sequence was aligned to AfAmt1 sequence using ClustalW [63] . Alignment was next submitted to Swiss-Model server [64] by using as template the AfAmt1 crystal (2B2H) [17] . The obtained structure was viewed and handled with PyMOL. How to cite this article : Boeckstaens, M. et al. The TORC1 effector kinase Npr1 fine tunes the inherent activity of the Mep2 ammonium transport protein. Nat. Commun. 5:3101 doi: 10.1038/ncomms4101 (2014).